Pseudogene-mediated posttranscriptional silencing of HMGA1 can result in insulin resistance and type 2 diabetes Processed pseudogenes are non-functional copies of normal genes that arise by a process of mRNA retrotransposition. The human genome contains thousands of pseudogenes; however, knowledge regarding their biological role is limited. Previously, we demonstrated that high mobility group A1 (HMGA1) protein regulates the insulin receptor ( INSR ) gene and that two diabetic patients demonstrated a marked destabilization of HMGA1 mRNA. In this paper we report that this destabilization of HMGA1 mRNA is triggered by enhanced expression of RNA from an HMGA1 pseudogene, HMGA1-p . Targeted knockdown of HMGA1-p mRNA in patient cells results in a reciprocal increase in HMGA1 mRNA stability and expression levels with a parallel correction in cell-surface INSR expression and insulin binding. These data provide evidence for a regulatory role of an expressed pseudogene in humans and establishes a novel mechanistic linkage between pseudogene HMGA1-p expression and type 2 diabetes mellitus. High mobility group A1 (HMGA1) is an architectural nuclear protein that binds to AT-rich regions of DNA and functions mainly as a specific cofactor for gene activation [1] , [2] . As part of an investigation into the molecular basis of regulation of the human INSR gene, we previously identified HMGA1 as a transcriptional regulator specifically needed for proper expression of this gene in eukaryotic mammalian cells [3] , [4] . Consistent with these findings, human type 2 diabetes (T2D) has been associated with defects in a nuclear regulatory protein either identical to, or highly related to, HMGA1, with commensurate decreases in INSR expression and consequent insulin resistance [3] , [4] , [5] . In this study, we report on two unrelated patients affected by insulin resistance and T2D in whom the expression of HMGA1 was markedly reduced and INSR gene transcription was considerably impaired as assessed in Epstein–Barr Virus (EBV)-transformed lymphoblasts of both subjects. Patient 1, a non-obese 45-year-old Italian man with the usual features of T2D, came to medical attention because of fasting hyperglycemia and hyperinsulinemia, in the absence of other disorders such as acromegaly or glucocorticoid excess. Patient 2, an 11-year-old Japanese boy, was diagnosed with T2D at 6 years of age and had the male form of type A insulin resistance with acanthosis nigricans. By investigating the molecular events underlying the impaired expression of HMGA1 in both diabetic individuals, we have previously identified a heterozygous single-nucleotide G deletion in the 3′-untranslated region (UTR) of the HMGA1 gene, which seemed to be linked to the accelerated degradation of HMGA1 mRNA in patients' cells [5] . However, when the mutant 3′-UTR was cloned into the 3′ position of a luciferase reporter gene and its expression was analysed in vitro in transient transfection assays, luciferase activity decreased by only 50% [5] , suggesting that this mutation, although potentially contributing to the loss of HMGA1 mRNA, was not fully sufficient to account for the observed large decline in HMGA1 mRNA stability in vivo in these subjects. Here, we report the overexpression of a novel HMGA1 pseudogene in both diabetic individuals. This HMGA1-p RNA effectively competes with HMGA1 3′-UTR for a critical RNA stability factor. In this manner, the pseudogene RNA triggers a marked destabilization of HMGA1 mRNA with consequent loss of INSR expression and generation of the insulin resistance phenotype. Overexpression of the HMGA1-p pseudogene in diabetic patients HMGA1 mRNA and protein abundances were determined in EBV-transformed lymphoblasts from diabetic patients and non-diabetic control subjects. In EBV-transformed lymphoblasts from both patients 1 and 2, HMGA1 mRNA and protein levels were markedly reduced compared with levels in non-diabetic controls ( Fig. 1a ). The decrease in HMGA1 expression in EBV-transformed lymphoblasts from patients 1 and 2 closely paralleled the decrease in INSR mRNA and protein levels. INSR mRNA and protein abundances were normal in EBV-transformed lymphoblasts from all T2D patients expressing normal levels of HMGA1 ( Fig. 1a ). The protein studies were carried out on nuclear extracts; HMGA1 protein was undetectable in cytoplasmic extracts of patient and control cells. To explore mechanism(s) of HMGA1 deficiency, we carried out studies of HMGA1 mRNA expression by combining conventional and real-time quantitative reverse transcription (RT)-PCR assays with cloning and sequencing strategies. Unexpectedly, the PCR analysis of HMGA1 mRNA revealed two distinct cDNA products ( Fig. 1b ). Sequencing analyses revealed that the smaller 1,773 bp fragment represented isoform 5 of HMGA1 mRNA, the gene of which mapped on chromosome 6 at 6p21. In contrast, the 1,873 bp fragment showed ∼ 93% homology with the known sequence of the HMGA1 mRNA and seemed to represent a novel processed pseudogene that we named HMGA1-p . Its sequence has been deposited in GeneBank (accession number AC005041) as part of chromosome 2, and its position seems to be compatible with a previously identified HMGA1 gene retrotransposed copy [6] . It is to be particularly noted that the level of HMGA1-p mRNA expression was significantly increased in both patients when compared with healthy controls and with 27 of unrelated T2D subjects with and without the G deletion above (including the two previously identified patients with a hemizygous deletion of the HMGA1 gene [5] ), whereas mRNA abundance of its homologous HMGA1 coding gene was markedly reduced ( Fig. 1b ). Moreover, as revealed by northern blot analysis of total RNA from cultured lymphoblasts of patients and controls, the HMGA1/HMGA1-p molecular ratio was considerably decreased in patients 1 and 2 ( Fig. 1b ). 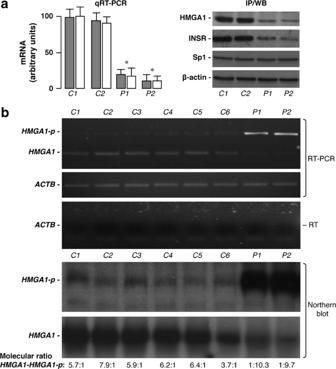Figure 1: HMGA1,HMGA1-pand INSR expression levels. (a) Comparison ofHMGA1mRNA (grey bars) and protein content withINSRmRNA (white bars) and protein expression in cultured lymphoblasts from controls (C1, C2) and patients (P1, P2). C1, representative of 20 normal subjects; C2, representative of 20 T2D patients with normal INSR expression. Normalized mRNA is expressed as a percentage of maximal value (100%). Results are the mean ± s.e.m. of three separate assays. *P<0.001 compared with controls. IP of the INSR and WB were performed using an anti-INSR β-subunit antibody. Sp1 and β-actin, control of nuclear and total cellular protein loading, respectively. (b)HMGA1andHMGA1-pmRNA as detected by a unique set of primers in semiquantitative RT–PCR of cDNA from cultured lymphoblasts of patients (P1, P2) and non-diabetic (C1-3, representative of 20 healthy subjects) and diabetic (C4-5, representative of 20 T2D patients) controls. mRNAs from T2D patients with the same G deletion as P1 and P2, but withoutHMGA1-poverexpression (C6, representative of seven T2D patients) are shown. Values were standardized withACTBmRNA. Genomic DNA contamination in RNA samples was excluded by PCR using aliquots of RNA without reverse transcription (−RT). Total RNA (5 μg) from the same set of cultured lymphoblasts was analysed by northern blot using cDNA probes forHMGA1andHMGA1-p. Representative autoradiograms are shown. Figure 1: HMGA1, HMGA1-p and INSR expression levels. ( a ) Comparison of HMGA1 mRNA (grey bars) and protein content with INSR mRNA (white bars) and protein expression in cultured lymphoblasts from controls (C1, C2) and patients (P1, P2). C1, representative of 20 normal subjects; C2, representative of 20 T2D patients with normal INSR expression. Normalized mRNA is expressed as a percentage of maximal value (100%). Results are the mean ± s.e.m. of three separate assays. * P <0.001 compared with controls. IP of the INSR and WB were performed using an anti-INSR β-subunit antibody. Sp1 and β-actin, control of nuclear and total cellular protein loading, respectively. ( b ) HMGA1 and HMGA1-p mRNA as detected by a unique set of primers in semiquantitative RT–PCR of cDNA from cultured lymphoblasts of patients (P1, P2) and non-diabetic (C1-3, representative of 20 healthy subjects) and diabetic (C4-5, representative of 20 T2D patients) controls. mRNAs from T2D patients with the same G deletion as P1 and P2, but without HMGA1-p overexpression (C6, representative of seven T2D patients) are shown. Values were standardized with ACTB mRNA. Genomic DNA contamination in RNA samples was excluded by PCR using aliquots of RNA without reverse transcription (−RT). Total RNA (5 μg) from the same set of cultured lymphoblasts was analysed by northern blot using cDNA probes for HMGA1 and HMGA1-p . Representative autoradiograms are shown. Full size image HMGA1-p affects HMGA1 mRNA and INSR expression and function The reciprocal relationship between HMGA1 and HMGA1-p mRNA suggested that overexpression of the HMGA1-p pseudogene may result in decreased HMGA1 protein expression, thereby leading to the observed decrease in INSR expression and the diabetic phenotype in these individuals. To test this model, a recombinant plasmid carrying the entire HMGA1-p pseudogene was generated and transiently transfected into cultured human HeLa cells, a cell line naturally expressing the homologous HMGA1 coding gene. As shown in Fig. 2a , treatment of HeLa cells with increasing amounts of HMGA1-p -containing plasmid caused a dose-dependent decrease in HMGA1 mRNA levels, with the maximal inhibition (50–60%) occurring at 2 μg recombinant vector. This reduction was specific for HMGA1 , as mRNA expression for the ubiquitously expressed transcription factor Sp1 was unaffected. Reduced HMGA1 mRNA levels paralleled the decrease in HMGA1 protein levels as detected by western blot (WB) analysis of nuclear extracts from transfected HeLa cells ( Fig. 2a ). Similar results were obtained in human HEK-293 cells, which do not express appreciable levels of endogenous HMGA1. As shown in Fig. 2a , HMGA1 mRNA and protein levels were impaired in HEK-293 cells when both HMGA1 and HMGA1-p were coexpressed simultaneously. When forced expression of HMGA1-p was induced in 3T3-L1 adipocytes (and in other insulin-sensitive human and mouse cell lines, such as HepG2 and Hepa-1 liver cell lines), HMGA1 and INSR expression levels were reduced, and this reduction was associated with a decrease in insulin signalling events, such as insulin-stimulated INSR β-subunit autophosphorylation and the phosphorylation of the insulin receptor substrate 1 (IRS1) ( Fig. 2b ). 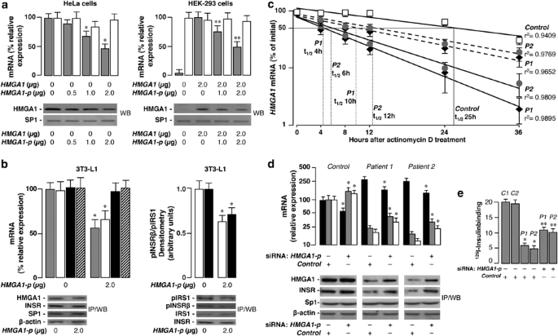Figure 2: Impact ofHMGA1-ponHMGA1mRNA levels and stability and on INSR expression and function. (a) HeLa and HEK-293 cells were transfected as indicated, andHMGA1(grey bars) and controlSp1(white bars) mRNA and protein levels were measured by real-time PCR and WB, respectively. mRNA is expressed as a percentage of max (100%, untransfected HeLa cells or HEK-293 cells plus HMGA1 alone). Results are the mean ± s.e.m. of three experiments. *P<0.05 versus untransfected HeLa cells; **P<0.05 versus HEK-293 cells overexpressing HMGA1 alone. (b) Left: HMGA1 (grey bars), INSR (white bars), Sp1 (black bars) and β-actin (slashed bars) mRNA and protein (IP/WB), as measured in 3T3-L1 adipocytes, before and after transfectingHMGA1-pexpression vector. Right: INSR and IRS1 expression and INSR β-subunit (pINSRβ) and IRS1 (pIRS1) phosphorylation were determined by IP/WB of insulin-stimulated lysates from untransfected and transfected cells. White bars, pINSRβ; black bars, pIRS1. Densitometric results are the mean ± s.e.m. Results are from three independent experiments. *P<0.05 versus untransfected 3T3-L1 cells. (c)HMGA1mRNA decay in patients and control cells treated with non-targeting siRNA (solid lines), orHMGA1-psiRNA (dashed lines). Open square, control (representative of 20 normal subjects); solid diamond, patient 1 (P1); solid circle, patient 2 (P2). mRNA amount at each time point is expressed as a percentage of max (100%, time 0), plotted on semilog axes. Results are the mean ± s.e.m. of triplicates from three independent experiments. (d)HMGA1-p(black bars),HMGA1(grey bars) andINSR(white bars) mRNA in cultured lymphoblasts from controls (n=20) and patients 1 and 2, after treatment with control/HMGA1-psiRNA. Results are means ± s.e.m. of three real-time PCRs. *P<0.05 versus untreated cells, per condition. HMGA1 and INSR protein levels are shown in representative IP/WB of three independent experiments. (e) Insulin binding to EBV-transformed lymphoblasts pretreated with control/HMGA1-psiRNA. Binding is expressed as percentage of total/107cells. Results are the mean ± s.e.m. of three separate experiments. C1, healthy subjects (n=20); C2, T2D patients with normal HMGA1 expression (n=20); P1 and P2, patients 1 and 2.*P<0.001 versus control (C1, C2) cells;**P<0.05 versus untreated patient's (P1, P2) cells. Figure 2: Impact of HMGA1-p on HMGA1 mRNA levels and stability and on INSR expression and function. ( a ) HeLa and HEK-293 cells were transfected as indicated, and HMGA1 (grey bars) and control Sp1 (white bars) mRNA and protein levels were measured by real-time PCR and WB, respectively. mRNA is expressed as a percentage of max (100%, untransfected HeLa cells or HEK-293 cells plus HMGA1 alone). Results are the mean ± s.e.m. of three experiments. * P <0.05 versus untransfected HeLa cells; ** P <0.05 versus HEK-293 cells overexpressing HMGA1 alone. ( b ) Left: HMGA1 (grey bars), INSR (white bars), Sp1 (black bars) and β-actin (slashed bars) mRNA and protein (IP/WB), as measured in 3T3-L1 adipocytes, before and after transfecting HMGA1-p expression vector. Right: INSR and IRS1 expression and INSR β-subunit (pINSRβ) and IRS1 (pIRS1) phosphorylation were determined by IP/WB of insulin-stimulated lysates from untransfected and transfected cells. White bars, pINSRβ; black bars, pIRS1. Densitometric results are the mean ± s.e.m. Results are from three independent experiments. * P <0.05 versus untransfected 3T3-L1 cells. ( c ) HMGA1 mRNA decay in patients and control cells treated with non-targeting siRNA (solid lines), or HMGA1-p siRNA (dashed lines). Open square, control (representative of 20 normal subjects); solid diamond, patient 1 (P1); solid circle, patient 2 (P2). mRNA amount at each time point is expressed as a percentage of max (100%, time 0), plotted on semilog axes. Results are the mean ± s.e.m. of triplicates from three independent experiments. ( d ) HMGA1-p (black bars), HMGA1 (grey bars) and INSR (white bars) mRNA in cultured lymphoblasts from controls ( n =20) and patients 1 and 2, after treatment with control/ HMGA1-p siRNA. Results are means ± s.e.m. of three real-time PCRs. * P <0.05 versus untreated cells, per condition. HMGA1 and INSR protein levels are shown in representative IP/WB of three independent experiments. ( e ) Insulin binding to EBV-transformed lymphoblasts pretreated with control/ HMGA1-p siRNA. Binding is expressed as percentage of total/10 7 cells. Results are the mean ± s.e.m. of three separate experiments. C1, healthy subjects ( n =20); C2, T2D patients with normal HMGA1 expression ( n =20); P1 and P2, patients 1 and 2. *P <0.001 versus control (C1, C2) cells; **P <0.05 versus untreated patient's (P1, P2) cells. Full size image Accumulating evidence strongly implicates posttranscriptional mechanisms involving mRNA structure (for example, folding) and mRNA stability in the regulation of gene expression [7] . To determine whether HMGA1-p overexpression in patients 1 and 2 was involved in posttranscriptional processes affecting HMGA1 expression, we examined the half-life of HMGA1 mRNA in the EBV-transformed lymphoblasts of patients. HMGA1 mRNA half-life decreased from ∼ 26 h in control cells to 4–6 h in cells of diabetic individuals overexpressing HMGA1-p ( Fig. 2c ). When studies of mRNA decay were conducted in patients' cells transfected with small interfering RNA (siRNA) specific to HMGA1-p , HMGA1 mRNA was stabilized, exhibiting a half-life of 10–12 h ( Fig. 2c ), along with a parallel increase in HMGA1 mRNA abundance ( Fig. 2d ). These data revealed an inverse correlation between HMGA1-p pseudogene expression and expression of its homologous HMGA1 coding gene in these individuals. Interestingly, the partial restoration of HMGA1 mRNA levels after treating cells with siRNA against HMGA1-p was accompanied by a concomitant increase in INSR mRNA and protein expression levels ( Fig. 2d ), and this increase was followed by a restoration of cell-surface insulin binding in patients' cells ( Fig. 2e ). The fact that transfection of patients' cells with siRNA to HMGA1-p significantly, but not completely, corrected HMGA1 mRNA stability and levels is consistent with the possibility that G deletion in the 3′-UTR of the HMGA1 gene, in these patients, can synergize with HMGA1-p overexpression in inducing HMGA1 mRNA destabilization/degradation. Impact of HMGA1-p 3′-UTR on HMGA1 mRNA expression To further explore the role of HMGA1-p in the control of HMGA1 mRNA stability, we mapped the segment of the HMGA1-p RNA that is critical to this pathway. Cells were transiently transfected with recombinant vectors carrying either the full-length or the truncated version of HMGA1-p . 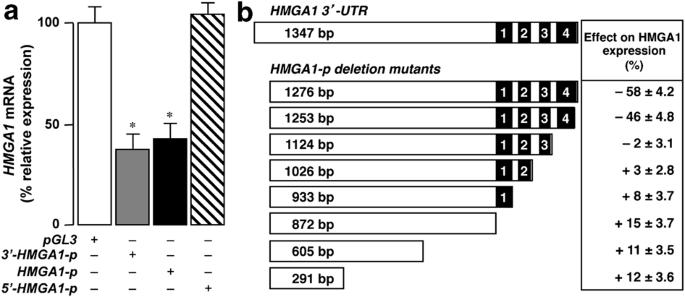Figure 3: Effects ofHMGA1-pand its derivatives on HMGA1 expression. (a)HMGA1mRNA was reduced in HeLa cells transfected with expression vectors containing the homologousHMGA1-p3′-UTR (grey bar) or the full-lengthHMGA1-p(black bar), and was unaffected in cells transfected with the expression vector containing the homologousHMGA1-p5′-UTR (dashed bar). The relative activity of pGL3 control vector alone was set at 100%. Results are the mean ± s.e.m. of three independent real-time PCRs.P<0.05 versus control. (b) Left: schematic representation ofHMGA13′-UTR and various deletion mutants of theHMGA1-phomologous region. Highly conserved regions (1–4) are highlighted in both 3′-UTR regions. Right: Effects of deletion mutants onHMGA1mRNA expression, as measured by real-time PCR in transfected HeLa cells. Results are the mean ± s.e.m. of three separate experiments. As shown in Figure 3a , transfection of HeLa cells with the recombinant plasmid HMGA1-p lacking the 248 bp 5′ region (corresponding to the 5′-UTR of HMGA1 gene) caused a 50% decrease in HMGA1 mRNA expression. This reduction was similar to the reduction obtained by transfecting full-length HMGA1-p . In contrast, no decrease in HMGA1 expression was observed in cells transfected with plasmid containing HMGA1-p lacking the 1,276 bp 3′ region (corresponding to the 3′-UTR of the HMGA1 gene) ( Fig. 3a ), suggesting that cis -acting element(s) in the 3′ region of HMGA1-p is (are) responsible for the observed impact on HMGA1 mRNA instability/degradation. This observation is consistent with our previous results indicating that HMGA1 3′-UTR has critical posttranscriptional regulatory elements within its 3′-UTR [8] . To characterize in greater detail those regions of the HMGA1-p 3′-UTR that were implicated in posttranscriptional processes affecting HMGA1 mRNA stability/degradation, several deletion mutants of HMGA1-p 3′-UTR, containing homologous regions of HMGA1 , were cloned into the pcDNA 3 plasmid vector, and analysed in transient transfection assays for their ability to interfere with transcription of the homologous HMGA1 gene. Real-time RT-PCR analysis revealed that the expression level of endogenous HMGA1 was only slightly increased in HeLa cells, in the presence of recombinant plasmids bearing proximal deletion mutants of HMGA1-p 3′-UTR (Δ291–Δ1026) ( Fig. 3b ). In contrast, HMGA1 mRNA abundance was considerably decreased in the presence of recombinant constructs containing the distal deletion mutants of HMGA1-p 3′-UTR (Δ1253 and Δ1276) ( Fig. 3b ). As shown in Fig. 3b , deletion of 152 bp of the 3′ end of the HMGA1-p 3′-UTR (region 4) reduced HMGA1 expression to approximately 40–50%, suggesting the presence, within this region, of elements that can decrease endogenous HMGA1 mRNA expression in trans . A possible mechanism for this control may be titration by HMGA1-p RNA of one or more trans -acting cytoplasmic protein factors critical to HMGA1 mRNA stability. Figure 3: Effects of HMGA1-p and its derivatives on HMGA1 expression. ( a ) HMGA1 mRNA was reduced in HeLa cells transfected with expression vectors containing the homologous HMGA1-p 3′-UTR (grey bar) or the full-length HMGA1-p (black bar), and was unaffected in cells transfected with the expression vector containing the homologous HMGA1-p 5′-UTR (dashed bar). The relative activity of pGL3 control vector alone was set at 100%. Results are the mean ± s.e.m. of three independent real-time PCRs. P <0.05 versus control. ( b ) Left: schematic representation of HMGA1 3′-UTR and various deletion mutants of the HMGA1-p homologous region. Highly conserved regions (1–4) are highlighted in both 3′-UTR regions. Right: Effects of deletion mutants on HMGA1 mRNA expression, as measured by real-time PCR in transfected HeLa cells. Results are the mean ± s.e.m. of three separate experiments. Full size image Physical association of αCP1 with the HMGA1 and HMGA1-p 3′-UTR To better understand the mechanism underlying the ability of HMGA1-p to reduce HMGA1 mRNA stability and induce HMGA1 mRNA degradation, we carried out a series of RNA-electrophoretic mobility shift assay (EMSA) combined with pull-down and immunoblot assays to identify the corresponding shared RNA-binding proteins. 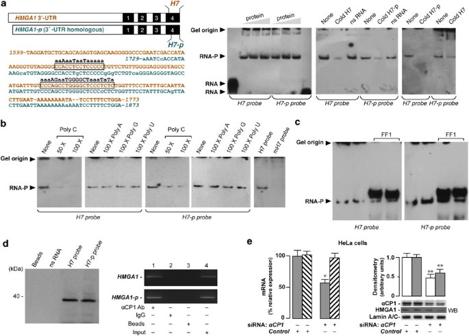Figure 4: mRNA–protein binding activity, physical association of αCP1 withHMGA1andHMGA1-p3′-UTR and αCP1 depletion. (a) Left: Localization and cDNA sequences of probes H7 (brown) and H7-p (green). C-rich elements targeting αCP1 are in boxes. Mutated C-rich elements of H7 are in black lowercase letters. Right: RNA-EMSAs showing binding of the α-complex family member(s) to either probe H7 or H7-p. HeLa protein extracts (2–6 μg, left panel) were incubated with either probe, and complexes resolved by EMSA. Sequence specificity of RNA-binding proteins was determined by using a 30-fold molar excess of unlabelled H7, H7-p or a nonspecific (ns) competitor RNA (centre panel). Labelled H7 or H7-p RNA was incubated with protein, in the absence or presence of a 30-fold molar excess of unlabelled H7-p or unlabelled H7, respectively, and cross-competition of H7 and H7-p was analysed (right panel). Free (RNA) and bound (RNA-P) probes are indicated in representative assays. (b) Effect of homoribopolymers poly(C), poly(A), poly (G), poly (U) and a mutated H7 (mH7) probe on EMSA. (c) In supershift assays, extracts were preincubated with the anti-αCP1 antibody (FF1 antiserum) before adding the probe. (d) RNA pull-down and RNA IP. Lysates were subjected to pull-down (left) in the presence of biotinylated H7, H7-p or nonspecific (ns) RNA probe, followed by WB with FF1 antiserum. RT-PCR was used for the detection ofHMGA1andHMGA1-pmRNA (right) in HeLa extracts following IP of αCP1 protein, using the FF1 antiserum. Co-immunoprecipitated RNA, as well as RNA present in an aliquot of the initial extracts, was subjected to RT–PCR (input). IP using rabbit IgG, used as negative control. (e) Effects of αCP1 depletion. HeLa cells were treated with anti-αCP1 siRNA (100 pmol) or a non-targeting control siRNA, and endogenousHMGA1mRNA (grey bars) was measured 48–96 h later by quantitative RT–PCR. In parallel experiments, HMGA1 protein expression was revealed by WB from HeLa extracts.Lamin A/CmRNA (dashed bars) and protein, used as controls. Representative WB is shown. Densitometric analyses of αCP1 (white bars) and HMGA1 (grey bars) WB are in bar graphs. Results are the mean ± s.e.m. of four separate assays.*P<0.05,HMGA1mRNA versus siRNA control;**P<0.05, αCP1 andHMGA1protein levels versus siRNA control. As shown in Figure 4a , RNA–protein binding activity was detected with both HMGA1 (H7) and HMGA1-p (H7-p) biotinylated 3′-UTR mRNA probes, in the presence of increasing amounts of cytoplasmic extracts from HeLa cells. To determine the specificity of RNA–protein binding, competition assays were performed. A 30-fold excess of either unlabelled H7 or unlabelled H7-p significantly reduced the binding of labelled H7 and labelled H7-p to the RNA-binding proteins, respectively, whereas the presence of the same amount of nonspecific competitor RNA had no significant effect on the complex formation ( Fig. 4a ). Moreover, unlabelled H7-p competitively inhibited the binding of labelled H7 to cytoplasmic proteins ( Fig. 4a ). In concert with this observation, unlabelled H7 inhibited the binding of labelled H7-p to cytoplasmic proteins ( Fig. 4a ). As this region of 3′-UTR mRNA contains three prominent and potentially important C-rich stretches, additional competition experiments were carried out with the synthetic homoribopolymer poly(C). Interaction of HeLa cytoplasmic proteins with either H7 or H7-p was markedly decreased in the presence of increasing amounts of poly(C) ( Fig. 4b ). This effect was specific, as no appreciable interference was detected in the presence of homoribopolymers poly(A), poly(G) or poly(U), and this specificity was further confirmed by lack of RNA–protein binding on incubation with the H7 probe in which mutations within the C-rich stretches were generated ( Fig. 4b ). On the basis of these observations, we hypothesized a role in RNA–protein binding activity for αCP proteins, a group of KH-domain RNA-binding proteins with binding specificity to C-rich patches, which have prominent roles in mRNA stability control [9] , [10] , [11] . Consistent with this hypothesis, the unique protein–RNA complex in HeLa cells was recognized and supershifted to a slower-migrating form by incubation with an affinity purified antiserum to the C-binding protein, αCP1 (FF1) ( Fig. 4c ). These data were substantiated by pull-down and RNA immunoprecipitation (IP) of αCP1–RNA complexes from HeLa cell extracts ( Fig. 4d ), suggesting that αCP1 binds in vivo , as well as in vitro , to HMGA1 and HMGA1-p RNAs. In agreement with these observations, HMGA1 mRNA and protein levels were decreased in HeLa cells following siRNA-mediated knockdown of endogenous αCP1 expression ( Fig. 4e ). Figure 4: mRNA–protein binding activity, physical association of αCP1 with HMGA1 and HMGA1-p 3′-UTR and αCP1 depletion. ( a ) Left: Localization and cDNA sequences of probes H7 (brown) and H7-p (green). C-rich elements targeting αCP1 are in boxes. Mutated C-rich elements of H7 are in black lowercase letters. Right: RNA-EMSAs showing binding of the α-complex family member(s) to either probe H7 or H7-p. HeLa protein extracts (2–6 μg, left panel) were incubated with either probe, and complexes resolved by EMSA. Sequence specificity of RNA-binding proteins was determined by using a 30-fold molar excess of unlabelled H7, H7-p or a nonspecific (ns) competitor RNA (centre panel). Labelled H7 or H7-p RNA was incubated with protein, in the absence or presence of a 30-fold molar excess of unlabelled H7-p or unlabelled H7, respectively, and cross-competition of H7 and H7-p was analysed (right panel). Free (RNA) and bound (RNA-P) probes are indicated in representative assays. ( b ) Effect of homoribopolymers poly(C), poly(A), poly (G), poly (U) and a mutated H7 (mH7) probe on EMSA. ( c ) In supershift assays, extracts were preincubated with the anti-αCP1 antibody (FF1 antiserum) before adding the probe. ( d ) RNA pull-down and RNA IP. Lysates were subjected to pull-down (left) in the presence of biotinylated H7, H7-p or nonspecific (ns) RNA probe, followed by WB with FF1 antiserum. RT-PCR was used for the detection of HMGA1 and HMGA1-p mRNA (right) in HeLa extracts following IP of αCP1 protein, using the FF1 antiserum. Co-immunoprecipitated RNA, as well as RNA present in an aliquot of the initial extracts, was subjected to RT–PCR (input). IP using rabbit IgG, used as negative control. ( e ) Effects of αCP1 depletion. HeLa cells were treated with anti-αCP1 siRNA (100 pmol) or a non-targeting control siRNA, and endogenous HMGA1 mRNA (grey bars) was measured 48–96 h later by quantitative RT–PCR. In parallel experiments, HMGA1 protein expression was revealed by WB from HeLa extracts. Lamin A/C mRNA (dashed bars) and protein, used as controls. Representative WB is shown. Densitometric analyses of αCP1 (white bars) and HMGA1 (grey bars) WB are in bar graphs. Results are the mean ± s.e.m. of four separate assays. *P <0.05, HMGA1 mRNA versus siRNA control; **P <0.05, αCP1 and HMGA1 protein levels versus siRNA control. Full size image Thus, we propose that by competing for the trans -acting cytoplasmic protein, αCP1, the overexpression of the HMGA1-p pseudogene RNA in affected individuals destabilizes HMGA1 mRNA with a corresponding decrease in HMGA1 protein production ( Fig. 5 ). The decrease in HMGA1 results in a corresponding decrease in INSR gene transcription, with consequent insulin resistance and T2D. 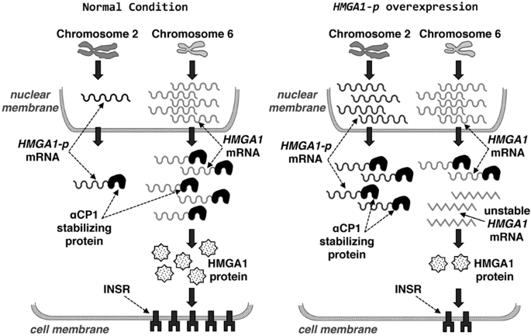Figure 5: Model for the role ofHMGA1-ppseudogene in diabetes. In the two individuals described in this report, abnormally high levels of theHMGA1-ppseudogene transcript are shown to compete withHMGA1mRNA for the RNA-binding protein αCP1. αCP1 normally stabilizesHMGA1mRNA on binding to a C-rich stability determinant in its 3′-UTR. By accelerating the degradation ofHMGA1mRNA,HMGA-1pRNA inhibits HMGA1 protein production with a consequent decrease inINSRgene transcription. The loss of INSR protein underlies the resultant insulin resistance and T2D in these two individuals. Figure 5: Model for the role of HMGA1-p pseudogene in diabetes. In the two individuals described in this report, abnormally high levels of the HMGA1-p pseudogene transcript are shown to compete with HMGA1 mRNA for the RNA-binding protein αCP1. αCP1 normally stabilizes HMGA1 mRNA on binding to a C-rich stability determinant in its 3′-UTR. By accelerating the degradation of HMGA1 mRNA, HMGA-1p RNA inhibits HMGA1 protein production with a consequent decrease in INSR gene transcription. The loss of INSR protein underlies the resultant insulin resistance and T2D in these two individuals. Full size image Processed pseudogenes result from reverse transcribed mRNAs [12] . In general, because pseudogenes lack promoters, they are no longer functional from the moment they are inserted into the genome and are not transcribed into mRNA [13] , [14] , [15] , [16] , [17] , [18] . However, recent evidence indicates that a subset of processed pseudogenes may perform regulatory functions. The ENCODE project has estimated that ∼ 20% of pseudogenes are transcribed with a pattern of tissue or cell line specificity [18] , [19] , and a number of functional pseudogenes have been shown to be indispensable for the evolution of mammals and can affect gene expression [20] , [21] . For example, it has been shown that, in Lymnea stagnalis , a pseudogene homologous to the nitric oxide synthase gene decreases the expression levels of his normal gene of origin through the formation of an RNA duplex that arises through a reverse-complement sequence found at the 5′ end of the pseudogene transcript [22] . In a second example, transcription of the makorin1-p1 pseudogene in mouse was required for the stability of mRNA from a homologous gene makorin1 [23] . Notwithstanding, this latter study has been subsequently challenged [24] , and a biological function for transcribed pseudogenes has been confirmed in several successive studies [25] , [26] , [27] , [28] , [29] , [30] . Despite multiple lines of evidence supporting functional role(s) of pseudogenes in mammals, evidence of a role of such interactions in human disease has heretofore been lacking. In this study, we describe a novel human HMGA1 pseudogene, HMGA1-p , which regulates mRNA stability of its corresponding coding gene. The data are consistent with a model by which the HMGA1-p pseudogene transcript effectively competes for a trans -acting cytoplasmic protein critical to the longevity of HMGA1 mRNA. By accelerating the degradation of HMGA1 mRNA transcript, the elevated levels of HMGA1-p RNA in affected individuals suppress expression of the INSR gene, resulting in insulin resistance and T2D. Previous studies have demonstrated that HMGA1 gene expression is posttranscriptionally regulated through signals within its 3′-UTR. Four highly conserved regions in this region seem to provide target-binding sites for RNA-binding proteins that are capable of either activating or inhibiting HMGA1 protein production [8] . Consistent with this observation, here we show that the ability of HMGA1-p to destabilize HMGA1 mRNA maps to the 3′ terminal portion of HMGA1-p mRNA. Remarkably, this region, which maintains extensive sequence homology with the HMGA1 3′-UTR, contains a series of three C-rich motifs. Such C-rich repeats have been previously linked to stabilization of a number of long-lived mRNAs [31] , [32] . By performing RNA–protein binding studies, we demonstrated that αCP1 interacts with either HMGA1 or HMGA1-p 3′-UTR and that cross-competition between the two RNA species for αCP1 can occur in both human and murine cells, in which increased levels of HMGA1-p transcript, by competing for the same trans -acting element involved in mRNA stabilization, may lead to increased HMGA1 mRNA degradation. The detrimental impact of HMGA1-p overexpression on HMGA1 mRNA expression was substantiated by siRNA knockdown of HMGA1-p in patient-derived lymphoblasts, in which the reduction in HMGA1-p transcript abundance was followed by a sustained increase in HMGA1 mRNA stability with an improvement in INSR expression and insulin-binding capacity. As αCP1 binds to many mRNA targets and no doubt affects their expression and metabolism, one might expect that the expression of HMGA1-p might have a pleiotropic effect. Thus, although the impact on HMGA1 mRNA and downstream INSR is clearly demonstrated in this paper, the apparent specificity of this effect remains an interesting observation that deserves further consideration. In conclusion, our findings further highlight the functional role of pseudogenes in the regulation of mRNA stability/degradation in mammals. In addition, the data provide the first direct evidence that overexpression of the HMGA1-p pseudogene can give rise to human-specific disorders such as T2D. Further studies can now be initiated to elucidate the mechanistic basis for the aberrant over­expression of HMGA1-p expression in affected individuals. Cells, IP/WB All experiments with human cells were approved by the Comitato Etico Regione Calabria, Azienda Ospedaleria 'Mater Domini', Catanzaro. EBV-transformed lymphoblasts were established from patients and from non-diabetic ( n =20) and diabetic ( n =27) individuals (Istituto G. Gaslini, Genova, Italy, Telethon Genetic Biobank Network, Project GTB07001A). All lymphoblastoid cell lines were maintained in RPMI 1640 medium supplemented with 15% fetal bovine serum and growth rates were similar in all cells. Human (HeLa and HEK-293) and mouse (3T3-L1) cell lines (ATCC) were maintained in Dulbecco's modified Eagle's medium with 10% fetal bovine serum. 3T3-L1 fibroblasts were differentiated into 3T3-L1 adipocytes according to a standard protocol [4] . In studies of insulin signalling, 3T3-L1 cells were serum deprived for 3 h and treated with insulin for 10 min before preparation of whole-cell lysates. IP and WB of INSR, HMGA1 and Sp1 were performed on total cellular lysates or nuclear extracts from EBV lymphoblasts and human and mouse cultured cells [3] , [4] . Total and tyrosine-phosphorylated INSR and IRS1 were assayed in 3T3-L1 cells after IP of cell lysates using INSRβ and IRS1 antibodies, followed by immunoblotting using an antiphosphotyrosine antibody. The antibodies used were anti-HMGA1 [3] , [4] ; anti-INSRβ, anti-Sp1, anti-β-actin (Santa Cruz Biotechnology); anti-phosphotyrosine and anti-IRS1 (Upstate Biotechnology). RT–PCR, northern blot, and mRNA decay Total cellular RNA was extracted from cells using an RNAqueous-4PCR kit and subjected to DNase treatment (Ambion). RNA levels were normalized against 18S ribosomal RNA in each sample. Complementary DNA was synthesized from total RNA with a RETROscript first strand synthesis kit (Ambion) and used for PCR amplification. Northern blots and hybridizations were carried out following standard procedures. Probes for HMGA1 and HMGA1-p were obtained by amplifying the respective 5′-UTR non-homologous regions. Hybridization signals were quantified with Molecular Dynamics PhosphorImager and Imagequant software (Molecular Dynamics). For the half-life of HMGA1 mRNA, logarithmic-phase EBV lymphoblasts were exposed to 0.5 μg ml −1 of actinomycin D. RNA was extracted at 4-h intervals, cDNA was prepared and HMGA1 mRNA levels were measured by quantitative RT-PCR, using RPS9 mRNA as control. mRNA half-life was determined by regression analysis and visual determination of the point at which the best-fit line crossed the 50% intercept. Transfections and 125 I-labelled insulin binding pGL3 control vector, containing HMGA1 or HMGA1-p , was transfected into either HeLa, HEK-293 or 3T3-L1 cells, using LipofectAMINE 2000 reagent (Invitrogen), and HMGA1 and INSR mRNA and protein expression levels were assayed 48–96 h later. For siRNA experiments, 100–200 pmol of siRNA targeted to HMGA1-p (Invitrogen) was transfected in EBV-transformed lymphoblasts (4×10 6 cells) using the diethylaminoethyl (DEAE) dextran method [4] , and nuclear extracts or total cellular lysates were prepared 72 h later. siRNA (100–200 pmol) was used to knock down αCP1 in transfected HeLa cells [33] . A nonspecific siRNA with a similar GC content (Dharmacon) and a non-targeting scrambled sequence (Santa Cruz Biotechnology) were used as a control. 125 I-insulin binding to EBV-transformed lymphoblasts treated with siRNA to HMGA1-p was measured 72 h after transfection [3] , [4] . EMSA and biotin pull-down assays The 3′ end of both HMGA1 (H7) and HMGA1-p (H7-p) cDNA containing the appropriate T7 promoter sequence was generated by PCR and 1 μg of PCR product was transcribed using the AmpliScribe T7-Flash Transcription Kit (Epicentre) with a portion of the UTP replaced by Biotin-16-UTP (Ambion). Biotin-labelled RNA probes (500 fmoles each) were incubated with HeLa cytoplasmatic extracts and RNA–protein binding and pull-down assays were performed. Briefly, the RNA probe was incubated for 1 h with protein extract (5 μg) in 1× binding buffer (10 mM Hepes, 40 mM KCl, 3.0 mM MgCl 2 , 1 mM dithiothreitol, 5% glycerol, 1 μg tRNA and 1.25 mg ml −1 heparin) at room temperature. The binding reaction was subsequently incubated with RNase A (10 ng μl −1 , Qiagen) for 10 min and 1 μl heparin (50 mg ml −1 ) was added to each reaction mixture. RNA–protein complexes were separated 10 min later on SDS–PAGE (6%) and transferred to Hybond-N+ membranes. Signal of RNA–protein binding was detected using the LightShift chemiluminescent kit (Pierce). FF1 antiserum antibody (against αCP1) [34] was used in supershift experiments. RNA used as nonspecific competitor was an oligonucleotide of unrelated sequence ( Supplementary Table S1 ) obtained by PCR using the AmpliScribe T7-Flash Transcription Kit, in the presence of T7 promoter sequence. RNA pull-down assays were carried out with 2 μg of either H7 or H7-p biotinylated probe coupled to Streptavidin-coated M280 Dynabeads (Invitrogen). HeLa cell lysates (100 μg) plus tRNA (50 μg) were added to RNA beads and incubated for 30 min at 4°C. At the end of the incubation period, the supernatant was removed, the beads were washed three times with 100 μl of hypotonic buffer, resuspended in 20 μl 1×Laemmli lysis buffer and analysed by WB analysis using FF1 antiserum. RNA IP assay HMGA1 mRNA was detected by RT–PCR, after RNA IP, using anti-αCP1 antibody FF1. HeLa cells (5×10 6 ) were lysed in IP buffer (50 mM Tris-HCl, pH 7.4/1% Nonidet P-40/0.5% sodium deoxycholate/0.05% SDS/1 mM EDTA/150 mM NaCl) containing protease inhibitors (Sigma) and 50 U ml −1 Superasin RNase inhibitor (Ambion), centrifuged at 12,000 g for 10 min at 4°C, after which the supernatant (0.75 ml) was added to 10 μg of FF1 antiserum antibody. After 2 h of incubation at room temperature, an equal volume of protein A/G agarose beads was added and the mixture was incubated for an additional 2 h. The protein A/G agarose–antibody–protein complexes were washed with IP buffer, bound RNAs were extracted using the RNAqueous-4PCR Kit and subjected to DNase treatment (Ambion); thereafter, HMGA1 mRNA was detected by RT–PCR. The studies on humans were approved by the local ethics committee (Comitato Etico Regione Calabria, Azienda Ospedaleria 'Mater Domini', Catanzaro). We obtained informed consent from all individuals or from their parents. Statistical analysis was performed using the Student's t -test. For all analyses, P <0.05 was considered significant. DNA and RNA sequences are described in Supplementary Table S1 . Accession numbers: HMGA1 mRNA variant 5: NM_145903 ; HMGA1-p : AC005041 ; HMGA1 mRNA variant 1: NM_145899 ; HMGA1 : NT_007592.15 . How to cite this article: Chiefari, E. et al . Pseudogene-mediated posttranscriptional silencing of HMGA1 can result in insulin resistance and type 2 diabetes. Nat. Commun. 1:40 doi: 10.1038/ncomms1040 (2010).